UPRmtscales mitochondrial network expansion with protein synthesis via mitochondrial import inCaenorhabditis elegans 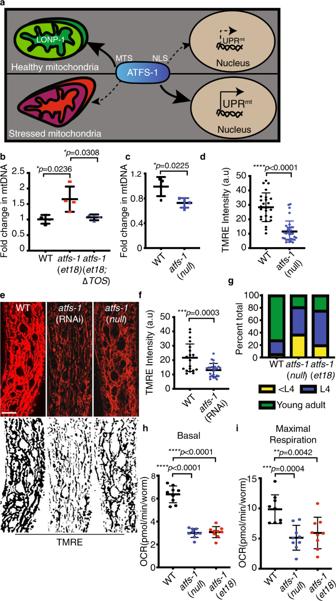Fig. 1: ATFS-1 regulates mitochondrial network expansion. aSchematic of ATFS-1 regulation.bQuantification of mtDNA in wild type,atfs-1(et18), andatfs-1(et18;ΔTOS)as determined by qPCR.N= 4 biologically independent experiments. Error bars mean ± SD (two-tailed Student’st-test).cQuantification of mtDNA in wild type andatfs-1(null).N= 4 biologically independent experiments. Error bars mean ± SD (two-tailed Student’st-test).dQuantification of TMRE intensity in the intestine of wild-type andatfs-1(null)worms. Experiments were repeated three biologically independent times with similar results.N= 21 worms (wild type),N= 33 worms((atfs-1(null)). Error bars mean ± SD (two-tailed Student’st-test). a.u. arbitrary units.eTMRE staining of wild-type worms raised on control oratfs-1(RNAi) andatfs-1(null)worms. Skeleton-like binary backbone is presented (bottom). Experiments were repeated three biologically independent times with similar results.N= 21 worms. Scale bar 10 µm.fQuantification of TMRE intensity in the intestine of wild-type andatfs-1(RNAi) worms. Experiments were repeated three biologically independent times with similar results.N= 25 worms. Error bars mean ± SD (two-tailed Student’st-test). a.u. Arbitrary units.gDevelopmental stages of 3-day-old wild-type,atfs-1(et18), oratfs-1(null)worms.N= 546 worms(wild type),N= 597 worms (atfs-1(et18)) and 627 worms (atfs-1(null)). Experiments were repeated two biologically independent times with similar results.h,iOxygen consumption rates (OCR) in wild type,atfs-1(et18), andatfs-1(null). Basal respiration (h), maximal respiration (i).N= 9 wells each containing ten worms. Error bars mean ± SD (two-tailed Student’st-test). Experiment was performed three biologically independent times with similar results. Source data are provided as a Source Data file. As organisms develop, individual cells generate mitochondria to fulfill physiological requirements. However, it remains unknown how mitochondrial network expansion is scaled to cell growth. The mitochondrial unfolded protein response (UPR mt ) is a signaling pathway mediated by the transcription factor ATFS-1 which harbors a mitochondrial targeting sequence (MTS). Here, using the model organism Caenorhabditis elegans we demonstrate that ATFS-1 mediates an adaptable mitochondrial network expansion program that is active throughout normal development. Mitochondrial network expansion requires the relatively inefficient MTS in ATFS-1, which allows the transcription factor to be responsive to parameters that impact protein import capacity of the mitochondrial network. Increasing the strength of the ATFS-1 MTS impairs UPR mt activity by increasing accumulation within mitochondria. Manipulations of TORC1 activity increase or decrease ATFS-1 activity in a manner that correlates with protein synthesis. Lastly, expression of mitochondrial-targeted GFP is sufficient to expand the muscle cell mitochondrial network in an ATFS-1-dependent manner. We propose that mitochondrial network expansion during development is an emergent property of the synthesis of highly expressed mitochondrial proteins that exclude ATFS-1 from mitochondrial import, causing UPR mt activation. Mitochondria are double-membrane bound organelles localized throughout the cytosol of eukaryotic cells; mitochondria are required for diverse essential activities including ATP production, nucleotide and amino acid synthesis, as well as serving as hubs for programmed cell death and innate immune signaling [1] . Mitochondria comprised ~1100 proteins [2] that are encoded by genes within the nuclear genome as well as within the mitochondrial genome (mtDNA) (12 in Caenorhabditis elegans ; 13 in mammals). Nuclear-encoded mitochondrial proteins are synthesized on cytosolic ribosomes and subsequently imported into mitochondria via a series of import channels and machineries [3] . Although much is known about mitochondrial biogenesis, it remains unclear how expansion of the mitochondrial network scales with cell growth in order to meet the physiological needs of each cell type. The UPR mt is a mitochondrial-to-nuclear signal transduction pathway regulated by the transcription factor ATFS-1, which is required for development and longevity during mitochondrial dysfunction [4] , [5] , [6] . As ATFS-1 harbors a mitochondrial targeting sequence (MTS) and a nuclear localization sequence (NLS), its transcription activity is regulated by subcellular localization. If ATFS-1 is imported into mitochondria, it is degraded by the protease LONP-1 [5] (Fig. 1a ). We previously showed that if a percentage of ATFS-1 fails to be imported into mitochondria, it traffics to the nucleus to activate a transcriptional response that includes mitochondrial chaperones [7] , [8] . Perturbations to oxidative phosphorylation (OXPHOS) or mitochondrial proteostasis activate the UPR mt as both processes are required for mitochondrial protein import [9] . In turn, ATFS-1 induces transcription to promote survival, and recovery from mitochondrial stress [10] . Fig. 1: ATFS-1 regulates mitochondrial network expansion. a Schematic of ATFS-1 regulation. b Quantification of mtDNA in wild type, atfs-1(et18) , and atfs-1(et18;ΔTOS) as determined by qPCR. N = 4 biologically independent experiments. Error bars mean ± SD (two-tailed Student’s t -test). c Quantification of mtDNA in wild type and atfs-1(null) . N = 4 biologically independent experiments. Error bars mean ± SD (two-tailed Student’s t -test). d Quantification of TMRE intensity in the intestine of wild-type and atfs-1(null) worms. Experiments were repeated three biologically independent times with similar results. N = 21 worms (wild type), N = 33 worms ((atfs-1(null)) . Error bars mean ± SD (two-tailed Student’s t -test). a.u. arbitrary units. e TMRE staining of wild-type worms raised on control or atfs-1 (RNAi) and atfs-1(null) worms. Skeleton-like binary backbone is presented (bottom). Experiments were repeated three biologically independent times with similar results. N = 21 worms. Scale bar 10 µm. f Quantification of TMRE intensity in the intestine of wild-type and atfs-1 (RNAi) worms. Experiments were repeated three biologically independent times with similar results. N = 25 worms. Error bars mean ± SD (two-tailed Student’s t -test). a.u. Arbitrary units. g Developmental stages of 3-day-old wild-type, atfs-1(et18) , or atfs-1(null) worms. N = 546 worms(wild type), N = 597 worms (atfs-1( et18 )) and 627 worms ( atfs-1(null) ). Experiments were repeated two biologically independent times with similar results. h , i Oxygen consumption rates (OCR) in wild type, atfs-1(et18) , and atfs-1(null) . Basal respiration ( h ), maximal respiration ( i ). N = 9 wells each containing ten worms. Error bars mean ± SD (two-tailed Student’s t -test). Experiment was performed three biologically independent times with similar results. Source data are provided as a Source Data file. Full size image Here we show that ATFS-1 and the UPR mt regulate an adaptable mitochondrial network expansion program that is active during C. elegans development. Worms lacking atfs- 1 have reduced expression of numerous genes required for mitochondrial biogenesis, relatively small mitochondria and fewer mtDNAs. Conversely, constitutive UPR mt activation results in increased mtDNA accumulation throughout development. We demonstrate that mitochondrial network expansion requires the weak MTS within ATFS-1, which allows the transcription factor to respond to reductions in mitochondrial protein import capacity. We find that impairment of S6 kinase results in impaired ATFS-1 activity due to mitochondrial accumulation of the transcription factor, while manipulations that increase TORC1-dependent protein synthesis activates the UPR mt , suggesting ATFS-1 responds to an increase in mitochondrial protein flux during development, to regulate mitochondrial network expansion. Consistent with this model, we demonstrate that over-expression of a single protein with a strong MTS is sufficient to expand the mitochondrial network in a manner dependent on ATFS-1. A role for ATFS-1 in mitochondrial network maintenance and expansion We previously found that deleterious mtDNA heteroplasmy resulted in an atfs-1 -dependent expansion of the mitochondrial network that was observed only when mitophagy was impaired [11] , suggesting a role for the UPR mt in mediating mitochondrial biogenesis. To gain further insights into the relationship between ATFS-1 and mitochondrial biogenesis during mitochondrial stress, we examined mtDNA accumulation in clk-1(qm30) worms, which lack a component required for ubiquinone biogenesis and activates the UPR mt [12] . clk-1(qm30) worms harbored more mtDNAs than wild-type worms, suggesting UPR mt activation leads to an increase in mtDNA quantity (Supplementary Fig. 1a ). atfs-1(et18) worms constitutively activate the UPR mt due to an amino acid substitution in the MTS, which impairs import into mitochondria even in the absence of mitochondrial stress [13] . Impressively, atfs-1(et18) worms harbored more mtDNAs relative to wild-type worms in both the L3 (Supplementary Fig. 1b ) and the L4 larval stages (Fig. 1b ), suggesting that UPR mt activation is sufficient to expand the mitochondrial network. Conversely, worms lacking the entire atfs-1 open reading frame ( atfs-1(null) ) [14] had reduced mtDNAs (Fig. 1c and Supplementary Fig. 1b ). Moreover, tetramethylrhodamine, ethyl ester (TMRE) staining indicated that atfs-1(null) or atfs-1 RNA interference (RNAi)-treated worms harbor fewer functional mitochondria relative to wild-type worms in intestinal cells (Fig. 1d–f ). Combined these findings suggest the UPR mt is actively involved in the maintenance and expansion of the mitochondrial network during development independent of exogenous mitochondrial stressors. atfs-1(null) worms developed slowly and had reduced respiration relative to wild-type worms (Fig. 1g–i ). atfs-1(et18) worms also developed slowly as previously documented [13] (Fig. 1g ). Surprisingly, despite the increased mtDNA quantity, atfs-1(et18) also respired less than wild-type worms (Fig. 1h, i ). The reduction in respiratory capacity in the atfs-1(et18) strain was consistent with reduced TMRE staining in intestinal cells (Supplementary Fig. 1c, d ). Thus, in the absence of the UPR mt , mtDNAs and functional mitochondrial are reduced, while continuous UPR mt activation results in a partial expansion of the mitochondrial network that yields dysfunctional mitochondria. ATFS-1 mediates a mitochondrial expansion program during development To elucidate the role of ATFS-1 in mitochondrial expansion and homeostasis, we compared transcriptional profiles of wild-type, atfs-1(null) , and atfs-1(et18 ) worms during development in the absence of mitochondrial stress. As expected, atfs-1(et18) worms induced mitochondrial genes including the proteostasis components associated with the UPR mt (Fig. 2a–d , Supplementary Fig. 2a–d , and Supplementary Data file 1 ). Furthermore, over 50 genes required for mitochondrial ribosome function were upregulated, as were genes required for mtDNA replication, and cardiolipin biosynthesis pathway genes that are essential for mitochondrial inner membrane synthesis. Lastly, genes required for both mitochondrial protein import and OXPHOS complex assembly were also upregulated. Fig. 2: ATFS-1 mediates a mitochondrial network expansion program. a Number of differentially regulated genes induced in atfs-1 ( et18 ) worms relative to wild type (WT) or reduce in atfs-1(null) worms relative to wild type. Green, upregulated; red, downregulated; and the number of overlapping genes between atfs-1(et18) and atfs-1(null) worms are listed in the last column. b – g Transcript levels of translation elongation factor mitochondrial 1 ( tsfm-1 ) and G elongation factor mitochondrial 1 ( gfm-1 ) ( b , e ), translocase of inner mitochondrial membrane 17B.1 ( timm-17B.1 ) and translocase of inner mitochondrial membrane-23 ( timm-23 ) ( c , f ), heat shock protein-6 ( hsp-6 ) and NADH:ubiquinone oxidoreductase complex assembly factor 3 ( nuaf-3 ) ( d , g ) as determined by qRT-PCR in wild type and atfs-1(et18) ( b – d ) or in wild type and atfs-1(null) ( e – g ). N = 3 biologically independent experiments except for gfm-1 ( e ) and nuaf-3 ( g ) N = 4. Error bars mean ± SD (two-tailed Student’s t -test). RFU, relative fluorescence units. h SDS-PAGE immunoblots of lysates from pdr-1(tm598 ), atfs-1(null);pdr-1(tm598) , and atfs-1(et18);pdr-1(tm598) worms. NDUFS3 is a component of the NADH:Ubiquinone Oxidoreductase complex I and tubulin (Tub) was used as a loading control. N = 3 biologically independent experiments with similar results. i – k . Transmission electron microscopy of body wall muscle of wild type ( i ), atfs-1(null) ( j ), and atfs-1(et18) worms ( k ). Scale bar 1 µm. Representative images from five worms analyzed from two biologically independent experiments with similar results. l Transmission electron microscopy of intestinal cells from wild-type, atfs-1(null) , and atfs-1(et18) worms. Mitochondria are highlighted in the middle panel. Scale bar 1 µm (left) and 200 nm (right). Representative images from five worms analyzed from two biologically independent experiments with similar results. Source data are provided as a Source Data file. Full size image Remarkably, most of the mitochondrial genes induced in the atfs-1(et18) strain were downregulated in the atfs-1(null) worms compared to wild-type worms (Figs. 2a, e–g , Supplementary Fig. 2b–d , and Supplementary Data files 2 and 3 ), consistent with less mtDNA and TMRE staining in intestinal cells (Fig. 1 ). Interestingly, the OXPHOS protein NDUFS3 was decreased in the atfs-1(null) worms, but unaffected in atfs-1(et18) worms (Fig. 2h and Supplementary Fig. 2e ), both of which are consistent with the RNA-sequencing (RNA-seq) data in each strain where the mRNA encoding the NDUFS3 transcript was reduced in atfs-1(null) worms and unchanged in atfs-1(et18) worms (Supplementary Data files 4 and 5 ). To exclude potential effects of mitochondrial degradation via mitophagy, these studies were performed in a strain lacking pdr-1 (Parkin) [15] . Interestingly, multiple mRNAs encoding tricarboxylic acid (TCA) cycle and OXPHOS components were repressed in atfs-1(et18) relative to wild-type worms (Supplementary Data file 5 ), consistent with our previous results where ATFS-1 limited transcription of highly expressed mitochondrial proteins during severe mitochondrial stress [8] . Lastly, although many mRNAs encoding mitochondrial proteins were expressed at lower levels in atfs-1(null) worms, mtDNA replication and mitophagy components were upregulated suggesting an alternative stress response(s) is induced in the absence of atfs-1 (Fig. 2a ). Because of the alterations in mtDNA levels, TMRE, and transcription of mitochondrial components in atfs-1 mutant worms, we visualized mitochondria via transmission electron microscopy. Impressively, mitochondria in atfs-1(null) worms were smaller and appeared defective in both intestine and muscle cells, along with pervasive muscle cell aberrations (Fig. 2i–l and Supplementary Fig. 2f ). In contrast, mitochondria in atfs-1(et18) worms were elongated, which was especially apparent in the intestine (Fig. 2i–l and Supplementary Fig. 2f ). As worms lacking atfs-1 harbor small and dysfunctional mitochondria, and atfs-1 is required for transcription of multiple genes required for mitochondrial biogenesis, our findings suggest that ATFS-1 regulates a mitochondrial expansion program. However, it should be considered that while ATFS-1 with an impaired MTS induces expression of mitochondrial biogenesis genes, it also impairs transcription of multiple TCA cycle and OXPHOS genes. These findings are similar to our previous results indicating that during severe mitochondrial dysfunction ATFS-1 bound the promoters of TCA cycle and OXPHOS genes and also limited their expression [8] . A weak MTS regulates ATFS-1, UPR mt , and mitochondrial network expansion We next sought to determine how ATFS-1 is regulated, or excluded from mitochondria, during development. As ATFS-1 harbors an MTS along with a NLS, we have proposed that the UPR mt is regulated by protein import capacity of the entire mitochondrial network [5] . ATFS-1 is predicted to have a relatively weak, or inefficient, MTS compared to other mitochondrial-targeted proteins such as mitochondrial chaperones and OXPHOS components [16] , [17] , [18] (Fig. 3a ). To compare the MTS strength of the OXPHOS protein ATP synthase subunit 9 (Su9) to ATFS-1, the N terminus of each was fused to green fluorescent protein (GFP) and expressed in HEK293T cells. As expected, both GFP-fusion proteins accumulated within mitochondria, but unlike Su9 (1-69) ::GFP, ATFS-1 (1-100) ::GFP fluorescence also accumulated within the cytosol, but to a lesser extent than that of ATFS-1 et18(1-100) ::GFP (Fig. 3b ). In addition, import of ATFS-1 (1-100) ::GFP was limited compared to Su9 (1-69) ::GFP in an in vitro import assay (Fig. 3d ), consistent with ATFS-1 harboring a weak MTS. Fig. 3: UPR mt requires the weak MTS in ATFS-1. a Mitochondrial targeting sequence probability prediction using MitoFates. OXPHOS proteins (red), mitochondrial chaperones (blue), ATFS-1 (black). b HEK293T cells expressing ATFS-1 1–100 ::GFP, ATFS-1 1-100(R/R) ::GFP, ATFS-1 1-100(et18) ::GFP or SU9 1–69 ::GFP. Scale bar 10 µm. Experiment was repeated two biologically independent times with similar results. c ATFS-1 schematic highlighting ATFS-1 R/R amino acid substitutions. d In organelle import of radiolabeled ATFS-1 1–100 ::GFP, ATFS-1 1-100(R/R) ::GFP and Su9 1–69 ::GFP into isolated mitochondria. After the indicated time points, mitochondria were washed and analyzed by SDS-PAGE electrophoresis. ATFS-1, Su9, mature (m) are marked. N = 3 biologically independent experiments with similar results. e SDS-Page immunoblots of lysates from wild-type, atfs-1 R/R , and atfs-1(et18) worms raised on control or lonp-1 (RNAi). ATFS-1 is marked (‣) and tubulin (Tub) was used as a loading control. N = 3 biologically independent experiments with similar results. f hsp-6 pr ::gfp in wild-type, atfs-1(et18) , and atfs-1 R/R worms. Scale bar 0.1 mm. N = 3 biologically independent experiments with similar results. g hsp-6 pr ::gfp in wild-type and atfs-1 R/R worms raised on 50 µg/ml EtBr, control, or timm-23 (RNAi). Scale bar 0.1 mm. N = 3 biologically independent experiments with similar results. h Developmental stages of 3-day-old wild-type or atfs-1 R/R worms. N = 158 worms (wild type) and N = 256 worms ( atfs-1 R/R ). Experiments were repeated two biologically independent with similar results. i TMRE staining of wild-type and atfs-1 R/R worms. Skeleton-like binary backbone is presented (right). Scale bar 10 µm. Experiments were repeated three times with similar results. j Quantification of mtDNA in wild-type and atfs-1 R/R worms as determined by qPCR. N = 3 biologically independent experiments. 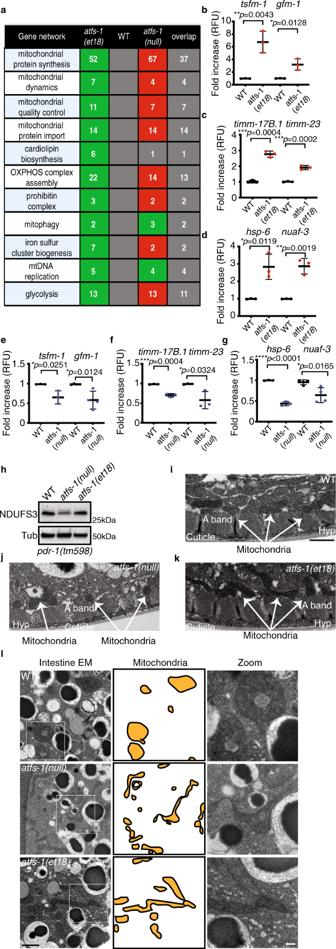Fig. 2: ATFS-1 mediates a mitochondrial network expansion program. aNumber of differentially regulated genes induced inatfs-1(et18) worms relative to wild type (WT) or reduce inatfs-1(null)worms relative to wild type. Green, upregulated; red, downregulated; and the number of overlapping genes betweenatfs-1(et18)andatfs-1(null)worms are listed in the last column.b–gTranscript levels of translation elongation factor mitochondrial 1 (tsfm-1) and G elongation factor mitochondrial 1 (gfm-1) (b,e), translocase of inner mitochondrial membrane 17B.1 (timm-17B.1) and translocase of inner mitochondrial membrane-23 (timm-23) (c,f), heat shock protein-6 (hsp-6) and NADH:ubiquinone oxidoreductase complex assembly factor 3 (nuaf-3) (d,g) as determined by qRT-PCR in wild type andatfs-1(et18)(b–d) or in wild type andatfs-1(null)(e–g).N= 3 biologically independent experiments except forgfm-1(e) andnuaf-3(g)N= 4. Error bars mean ± SD (two-tailed Student’st-test). RFU, relative fluorescence units.hSDS-PAGE immunoblots of lysates frompdr-1(tm598),atfs-1(null);pdr-1(tm598), andatfs-1(et18);pdr-1(tm598)worms. NDUFS3 is a component of the NADH:Ubiquinone Oxidoreductase complex I and tubulin (Tub) was used as a loading control.N= 3 biologically independent experiments with similar results.i–k. Transmission electron microscopy of body wall muscle of wild type (i),atfs-1(null)(j), andatfs-1(et18)worms (k). Scale bar 1 µm. Representative images from five worms analyzed from two biologically independent experiments with similar results.lTransmission electron microscopy of intestinal cells from wild-type,atfs-1(null), andatfs-1(et18)worms. Mitochondria are highlighted in the middle panel. Scale bar 1 µm (left) and 200 nm (right). Representative images from five worms analyzed from two biologically independent experiments with similar results. Source data are provided as a Source Data file. Error bars mean ± SD (two-tailed Student’s t -test). k Proposed model for ATFS-1-mediated mitochondria expansion. Source data are provided as a Source Data file. Full size image We hypothesized that the inefficient MTS allows ATFS-1 import and UPR mt activation to be sensitized to conditions that impact mitochondrial import capacity including mitochondrial stress, total mitochondria, and potentially the flux of other proteins into mitochondria. Thus, we sought to generate a worm strain expressing ATFS-1 with a stronger, or more efficient, MTS. Amino acid substitutions of T10 and D24 to arginine are predicted to increase MTS strength [16] (Fig. 3a, c ). Similar to Su9 (1-69) ::GFP, ATFS-1 R/R(1-100) ::GFP only accumulated within mitochondria and not in the cytosol in HEK293T cells (Fig. 3b ). Furthermore, more ATFS-1 R/R(1-100) ::GFP accumulated within mitochondria than ATFS-1 (1-100) ::GFP in an in vitro import assay, consistent with increased MTS strength (Fig. 3d ). Via CRISPR-Cas9, mutations were introduced at the endogenous atfs- 1 locus to generate atfs-1 R/R . We first examined accumulation of ATFS-1 R/R within mitochondria during normal development by raising worms on lonp-1 (RNAi), which impairs ATFS-1 degradation within the matrix [5] . Strikingly, more ATFS-1 R/R accumulated within mitochondria compared to wild-type ATFS-1 or ATFS-1 et18 during normal development (Fig. 3e ). ATFS-1 R/R worms had reduced hsp-6 pr ::gfp fluorescence relative to wild-type or atfs-1(et18) worms during normal development (Fig. 3f and Supplementary Fig. 3a ) and also had reduced expression of hsp-6 and timm-23 mRNAs (Supplementary Fig. 3b, c ). ATFS-1 R/R also impaired UPR mt activation caused by ethidium bromide (EtBr) exposure (Fig. 3g and Supplementary Fig. 3d ). However, timm-23 (RNAi), which impairs a component required for import of most proteins harboring N-terminal MTSs [9] , caused UPR mt activation in both ATFS-1 R/R and wild-type worms (Fig. 3g and Supplementary Fig. 3d ), indicating ATFS-1 R/R is a functional transcription factor likely impaired due to increased mitochondrial accumulation. Similar to worms lacking atfs-1 , worms expressing ATFS-1 R/R developed slower (Fig. 3h ) and exhibited a perturbed and fragmented mitochondrial network in both intestine and muscle cells along with a reduction in mtDNAs (Fig. 3i, j and Supplementary Fig. 3e–g ). Combined, these data suggest that ATFS-1 regulates a transcriptional program to expand mitochondrial biomass that is active throughout development and reliant on an inefficient MTS that confers sensitivity to conditions that impact mitochondrial import capacity. These findings suggest that during development a percentage of ATFS-1 cannot be imported into mitochondria of growing cells resulting in modest UPR mt activation and mitochondrial network expansion (Fig. 3k ). Interplay between components that regulate protein synthesis, mitochondrial import, and ATFS-1 Previous screens for components required for UPR mt activation identified multiple regulators of growth-related protein synthesis including the insulin-like receptor daf-2 , rheb-1 , mTOR ( let-363) , and rsks-1 (S6 kinase) [12] , [19] . TORC1 regulates protein synthesis rates in response to diverse inputs including growth signals and cellular energetics [20] . Insulin-like signaling-TORC1 promotes protein synthesis by phosphorylating RSKS-1, which in turn, phosphorylates a ribosomal subunit [20] (Supplementary Fig. 4a ). Alternatively, the 5′-AMP-activated protein kinase (AMPK) limits TORC1 activity and protein synthesis when ATP levels are low [21] , [22] . As expected, DAF-2 inhibition impaired induction of hsp-6 pr ::gfp (Supplementary Fig. 4b ) [23] . Furthermore, hsp-6, atfs-1 , the mitochondrial elongation factors gfm-1 , tsfm-1 , and timm-17 mRNAs were also reduced during normal development and during mitochondrial stress (Supplementary Fig. 4c–g ) similar to what was observed in atfs-1(null) worms. Inhibition of TORC1 components rheb-1 , raga-1 , mTOR , and rsks-1 also reduced hsp-6 pr ::gfp (Supplementary Fig. 4h–j ), as well as hsp-6 and atfs-1 , gfm-1 , tsfm-1 , and timm-17 mRNA levels, as did starvation (Fig. 4a, b and Supplementary Fig. 4k–p ). Conversely, inhibition of AMPK, which increases TORC1 activity, resulted in increased hsp-6 mRNA in an atfs-1 and mTOR -dependent manner (Fig. 4c–e ), whereas AMPK activation [24] reduced hsp-6 transcripts (Fig. 4f ). Moreover, AMPK inhibition resulted in increased binding of ATFS-1 to the hsp-6 promoter, suggesting increased nuclear localization of ATFS-1. Alternatively, the promoter occupancy of hsp-6 by ATFS-1 was reduced in the rsks-1(ok1255) worms relative to wild-type worms (Fig. 4g ). Combined, our results indicate that TORC1 and RSKS-1 are required for UPR mt during development and suggest that the relatively high level of protein synthesis during development stimulates UPR mt activity. Fig. 4: TORC1-mediated protein synthesis promotes ATFS-1 activation. a , b Transcript levels of heat shock protein-6 ( hsp-6 ) ( a ) and of activated transcription factor stress-1 ( atfs-1 ) ( b ) as determined by qRT-PCR in wild-type and rsks-1(ok1255) worms. N = 4 biologically independent experiments. Error bars mean ± SD (two-tailed Student’s t -test). RFU, relative fluorescence units. c hsp-6 pr ::gfp and aak-2(rr48);hsp-6 pr ::gfp worms raised on control, let-363 , or atfs-1 (RNAi). Scale bar 0.1 mm. Experiments were repeated three biologically independent times with similar results. d Quantification of GFP intensity in hsp-6 pr ::gfp ( N = 10) and aak-2(rr48);hsp-6 pr ::gfp worms raised on control ( N = 8 worms), let-363 ( N = 8 worms), or atfs-1 (RNAi) ( N = 7 worms). Error bars mean ± SD (two-tailed Student’s t -test). a.u., arbitrary units. e , f Transcript levels of heat shock protein-6 ( hsp-6 ) as determined by qRT-PCR in wild-type and aak-2(rr48) worms N = 3 biologically independent experiments ( e ) and in wild type, agd383 , and agd383;atfs-1(et18) strains N = 5 biologically independent experiments ( f ). Error bars mean ± SD (two-tailed Student’s t -test). RFU, relative fluorescence units. g ChIP of hsp-6 promoter in wild-type, rsks-1(ok1255) , and aak-2(rr48) worms as measured by qRT-PCR. N = 2 biologically independent experiments. RFU, relative fluorescence units. h SDS-Page immunoblots of wild-type and rsks-1(ok1255) worms, raised on control or lonp-1 (RNAi). Tubulin (Tub) was used as a loading control. N = 3 biologically independent experiments with similar results. i atfs-1(et18);hsp-6 pr ::gfp worms raised on control or rsks-1 (RNAi). Scale bar 0.1 mm. Experiments were repeated three biologically independent times with similar results. j TMRE staining (red) of worms expressing myo-3 pr ::gfp or myo-3 pr :: mt gfp . Scale bar 10 µm. Experiments were repeated three biologically independent times with similar results. k Quantification of TMRE intensity in muscle cells of worms expressing myo-3 pr ::gfp or myo-3 pr :: mt gfp . N = 34 worms ( myo-3 pr :: gfp ), N = 24 worms ( myo-3 pr :: mt gfp) . Error bars mean ± SD (two-tailed Student’s t -test). a.u., arbitrary units. l Quantification of mtDNA in myo-3 pr :: gfp and myo-3 pr :: mt gfp worms as determined by qPCR. N = 6 biologically independent experiments. Error bars mean ± SD (two-tailed Student’s t -test). m , n Transcript levels of translocase of inner mitochondrial membrane-23 ( timm-23 ) ( m ) and of heat shock protein-6 ( hsp-6 ) ( n ) as determined by qRT-PCR in myo-3 pr ::gfp and in myo-3 pr :: mt gfp worms. N = 4 biologically independent experiments. Error bars mean ± SD (two-tailed Student’s t -test). RFU, relative fluorescence units. o TMRE staining of worms expressing myo-3 pr :: mt gfp raised on control or atfs-1 (RNAi). Scale bar 10 µm. Experiments were repeated three biologically independent times with similar results. p Quantification of TMRE intensity in muscle cells of worms expressing myo-3 pr :: mt gfp raised on control or atfs-1 (RNAi). N = 18 worms (control), N = 13 worms ( atfs-1 (RNAi)). Error bars mean ± SD (two-tailed Student’s t -test). a.u., arbitrary units. q TMRE staining of wild-type and atfs-1 ( null ) worms expressing myo-3 pr :: mt gfp . Scale bar 10 µm. Experiments were repeated three biologically independent times with similar results. r Quantification of TMRE intensity in muscle cells of wild-type, and atfs-1(null) worms. N = 15 worms (wild type), N = 24 worms ( atfs-1(null) ). Error bars mean ± SD (two-tailed Student’s t -test). a.u., arbitrary units. s TMRE staining of wild-type and atfs-1 R/R worms expressing myo-3 pr :: mt gfp . Scale bar 10 µm. Experiments were repeated three biologically independent times with similar results. Source data are provided as a Source Data file. Full size image In mammals, TORC1 promotes protein synthesis by phosphorylating S6 kinase and 4EBP, which requires a TOR signaling (TOS) motif in each protein [25] . Interestingly, ATFS-1 also harbors a canonical TOS motif (-FEMDI-) (Fig. 3c ), which we mutated at the endogenous locus to yield -AEMDI- ( atfs-1(∆TOS) ). UPR mt activation was attenuated in atfs-1(∆TOS) worms relative to wild-type worms upon EtBr exposure (Supplementary Fig. 4q ). Importantly, the TOS motif was also required for the increased hsp-6 pr ::gfp (Supplementary Fig. 4r ) and mtDNA (Fig. 1b ) in atfs-1(et18) worms suggesting the TOS motif promotes nuclear function of ATFS-1, similar to the TOS motif found in the transcription factor HIF-1α [26] . Interestingly, hsp-6 pr ::gfp induction caused by EtBr or complex III-deficiency ( isp-1(qm150) [27] ), was impaired further in rsks-1(ok1255);atfs-1(∆TOS) worms relative to either atfs-1(∆TOS) or rsks-1(ok1255) worms (Supplementary Fig. 4s–u ), suggesting that RSKS-1 promotes UPR mt activation independent of the TOS motif. We examined the effect of rsks-1 inhibition on expression and trafficking of ATFS-1. One possibility is that rsks-1 inhibition simply reduces synthesis of ATFS-1 limiting its nuclear transcription activity. rsks-1(ok1255) worms had reduced atfs-1 mRNA relative to wild-type worms (Fig. 4b ). However, more ATFS-1 protein accumulated within mitochondria in rsks-1(ok1255) worms relative to wild-type worms (Fig. 4h ) suggesting UPR mt impairment in worms lacking RSKS-1 is due to mitochondrial accumulation of ATFS-1, similar to ATFS-1 R/R (Fig. 3e ). Importantly, rsks-1 (RNAi) did not reduce hsp-6 pr ::gfp in atfs-1(et18) worms with an impaired MTS (Fig. 4i ) or when treated with timm-23 (RNAi) (Supplementary Fig. 4v ). Lastly, increased hsp-6 pr ::gfp persisted during starvation in both atfs-1(et18) worms and timm-23 (RNAi) treated worms (Supplementary Fig. 4w, x ). Combined, these findings suggest that the reduced atfs-1 transcription in rsks- 1-mutant worms is not the cause of impaired UPR mt activation, rather the accumulation of ATFS-1 within mitochondria impairs atfs-1- dependent transcription. As RSKS-1 is required for protein synthesis during cell growth, we hypothesized that the high rate of mitochondrial protein import during development may cause UPR mt activation and mitochondrial network expansion. Interestingly, OXPHOS transcripts are among the most highly expressed mRNAs in worms (Supplementary Fig. 5a ). In addition, C. elegans ribosome profiling data indicate that OXPHOS proteins are translated primarily during the early stages of worm development (L1,L2), and are reduced or absent by the L4 stage (Supplementary Fig. 5b ). Interestingly, the ATFS-1 ribosome profile mirrors the OXPHOS profiles early in development and is also diminished at L4 (Supplementary Fig. 5c ), consistent with the observation that the UPR mt can only be activated by stress prior to the L4 stage [28] . Thus, we hypothesize that because of a weak MTS, a percentage of ATFS-1 is excluded from mitochondria during development by highly expressed mitochondrial proteins with stronger MTSs. As a test of this model, we sought to determine the impact of overexpressing a single protein with a relatively strong MTS on the mitochondrial network. The mitochondrial network was examined in muscle cells of worms expressing GFP or mt GFP via the strong myo-3 promoter [29] . Importantly, mt GFP harbors a relatively strong MTS (aa 1–24) from the enzyme aspartate aminotransferase (AST) (Supplementary Fig. 6a ) and the myo-3 promoter is expressed throughout development [30] (Supplementary Fig. 6b ). Strikingly, mt GFP expression increased accumulation of functional mitochondria as determined by TMRE staining (Fig. 4j, k ), mtDNA number (Fig. 4l ), and hsp-6 , timm-17 and timm-23 mRNAs (Fig. 4m–n and Supplementary Fig. 6c ) despite mt GFP being expressed at a lower level than GFP (Supplementary Fig. 6d, e ). Expansion of TMRE staining by mt GFP was impaired by atfs-1 (RNAi) (Fig. 4o, p ), atfs-1(null) (Fig. 4q, r ), and in ATFS-1 R/R worms (Fig. 4s ); however mt GFP transcription was not affected by the atfs-1(null) allele (Supplementary Fig. 6f ). To determine whether the mitochondrial network expansion caused by expression of mt GFP required nuclear trafficking of ATFS-1, we used CRISPR-Cas9 to introduce an amino acid substitution to perturb the NLS in ATFS-1 (R426A). atfs-1 ∆NLS worms were unable to induce hsp-6 pr ::gfp or endogenous hsp-6 transcripts during mitochondrial stress caused by spg-7 (RNAi) consistent with impaired nuclear activity (Supplementary Fig. 6g, h ). When raised on lonp- 1(RNAi), ATFS-1 (∆NLS) accumulated within mitochondria like wild-type ATFS-1 (Supplementary Fig. 6i ), indicating ATFS-1 ∆NLS was expressed and processed similarly to wild-type ATFS-1. The atfs-1 ∆NLS allele was crossed into myo-3 pr :: mt GFP worms to examine the effect on mitochondrial network expansion during development. Similar to atfs-1 R/R and atfs-1(null) worms, atfs-1 ∆NLS worms had a severely perturbed mitochondrial network in muscle cells as determined by TMRE staining (Supplementary Fig. 6j ). Thus, the NLS within ATFS-1 is essential for mitochondrial network expansion caused by expression of mt GFP. Combined, these findings indicate that expression of a single protein with a strong MTS is sufficient to expand the mitochondrial network in an atfs-1 -dependent manner. The UPR mt was discovered as a protective transcriptional response to unfolded protein accumulation within the mitochondria and OXPHOS perturbation [5] , [31] , [32] , [33] . Here, we demonstrate that ATFS-1 regulates a mitochondrial biogenesis or network expansion program that is basally active throughout normal development, which can be further activated by diverse mitochondrial perturbations. Developmental mitochondrial expansion required the inefficient MTS of ATFS-1, mTOR, and S6 kinase, suggesting an interplay between protein synthesis, mitochondrial protein import capacity, and nuclear activity of ATFS-1. We propose a model where the high levels of mitochondrial protein synthesis that occurs during development drives mitochondrial network expansion by excluding a percentage of ATFS-1 from mitochondrial import. In addition, network expansion continues until mitochondrial import capacity is sufficient to import ATFS-1 and terminate the UPR mt . These findings are conceptually similar to the endoplasmic reticulum expansion that occurs in response to increased protein flux via the UPR ER , which is regulated by IRE1 and XBP1 [34] . We propose that as a function of mitochondrial import flux or mitochondrial protein processing, ATFS-1 scales mitochondrial network expansion with cell growth. Intriguingly, it was recently reported that mitochondrial metabolic proteins are prone to stalling within mitochondrial import channels under basal conditions in growing cells [35] , [36] , suggesting import or intra-mitochondrial protein processing can be overwhelmed during normal cell growth, which may result in ATFS-1 activation. We previously found that during severe mitochondrial dysfunction ATFS-1 binds the promoters of many of the genes regulated by ATFS-1 during normal development including mitochondrial chaperones, mitochondrial protein import machinery, as well as mitochondrial ribosome component encoding genes. Intriguingly, the ATFS-1 chromatin immunoprecipitation (ChIP)-sequencing experiment also revealed that ATFS-1 bound the promoters many OXPHOS and TCA cycle genes. Surprisingly, ATFS-1 repressed or limited transcription of the OXPHOS and TCA cycle genes during mitochondrial stress. We suggested that repression of OXPHOS and TCA cycle transcription reduced the load of unfolded proteins in an already stressed mitochondria potentially allowing time for recovery [8] . Ribosome profiling indicates that during normal development, the highly expressed OXPHOS proteins are translated during the L1–L2 developmental stages and mostly reduced by the L4 stage [30] . We suggest that it is the expression of these and other mitochondrial proteins that leads to developmental activation of ATFS-1 by limiting the mitochondrial import of ATFS-1, resulting in mitochondrial network expansion. Consistent with this model, expression of mt GFP was sufficient to expand the muscle cell mitochondrial network in an atfs-1 -dependent manner (Fig. 4j–s ). If the mitochondrial network becomes perturbed during growth, reducing transcription of the most highly expressed substrates may prevent further damage and allow time for recovery. These insights potentially inform on the discrepancies between atfs-1(null) worms and atfs-1(et18) worms where despite having increased mtDNAs and mitochondrial biogenesis machinery transcripts, the mitochondrial network in atfs-1(et18) worms is dysfunctional (Supplementary Fig. 1c, d ). However, RNA-seq indicates that multiple TCA cycle and OXPHOS components are reduced in atfs-1(et18) worms relative to wild-type worms (Supplementary Data file 5 ). It is important to note that the atfs-1(et18) allele was isolated in a screen to identify mutations that confer resistance to high levels of statins [13] . Although the processes affected in atfs-1(et18) worms that confer statin resistance are unknown, the strain develops slowly and has a shortened lifespan relative to wild-type worms [13] . One potential reason is that in the atfs-1(et18) strain, ATFS-1 is not regulated by mitochondrial import capacity and remains constitutively active where in addition to increasing numerous genes that promote mitochondrial biogenesis also represses OXPHOS and TCA cycle component transcription. This uncoupling, or deregulation, may result in the generation of defective mitochondria. In conclusion, we propose that ATFS-1 responds to the high levels of mitochondrial protein import that occur during development. The relatively inefficient MTS of ATFS-1 matches insulin receptor (DAF-2) and S6 kinase-dependent synthesis of mitochondrial proteins to a transcriptional program that expands the mitochondrial network effectively scaling mitochondrial biogenesis with cell growth. However, if mitochondrial function is perturbed, ATFS-1 mitochondrial import is further perturbed causing additional nuclear accumulation where it reduces transcription of OXPHOS and TCA cycle components [8] reducing the burden on the mitochondrial protein folding and complex assembly machinery. Upon network recovery, developmental mitochondrial network expansion continues until mitochondrial protein import capacity is sufficient to import ATFS-1. Worms, plasmids, and staining The reporter strain hsp-6 pr ::gfp for visualizing UPR mt , and the myo-3 pr ::gfp and the myo-3 pr :: mt gfp for visualization of mitochondrial mass and atfs-1(null) worms have been previously described [14] , [32] , [33] . The MTS in the myo-3 pr :: mt gfp is the first 24 amino acids from the enzyme AST from Coturnix japonica (1-MALLQSRLLLSAPRRAAATARASS-24) fused to GFP. The atfs-1(et18) strain was a gift from Marc Pilon. N2(wild type), isp-1(qm150) , rsks-1(ok1255) , and daf-2(e1370) were obtained from the Caenorhabditis Genetics Center (Minneapolis, MN). The atfs-1 R/R ( cmh16 ), the atfs-1(∆TOS) ( cmh17 ), and the atfs-1(∆NLS)(cmh18) strains were generated via CRISPR-Cas9 in hsp-6 pr ::gfp worms as described [14] . The atfs-1(∆TOS) was generated in both the wild-type worms as well as in the atfs-1(et18) strain. The crRNAs (IDT) were co-injected with purified Cas9 protein, tracrRNA (Dharmacon), repair templates (IDT), and the pRF4::rol-6(su1006) plasmid as described [37] , [38] . The crRNAs and repair templates used in this study are listed in Supplementary Data file 6 . The pRF4::rol-6 (su1006) plasmid was a gift from Craig Mello [39] . The ATFS-1 1–100 ::GFP expressing plasmid was previously described [5] . The ATFS-1 1-100(R4C) ::GFP and the ATFS-1 1-100(T10R, D24R) ::GFP were generated by introducing mutations to yield the described amino acid substitutions in the ATFS-1 1–100 ::GFP expressing plasmid. The Su9 of the F0-ATPase (SU9) 1–69 ::GFP PQCXIP expression plasmid was a gift from Xuejun Jiang. Worms were raised HT115 strain of Escherichia coli and RNAi performed as described [40] . EtBr and TMRE experiments were performed by synchronizing and raising worms on plates previously soaked with M9 buffer containing EtBr or 2 µM TMRE. Worms were analyzed at the L4 larvae stage except for EtBr-treated worms that led to developmental arrest. EtBr-treated worms were analyzed at the same time as the control. Protein analysis and antibodies Synchronized worms were raised on plates with control(RNAi) or lonp-1 (RNAi) to the L4 stage prior to harvesting. Whole worm lysate preparation was previously described [33] . Antibodies against α-tubulin were purchased from Calbiochem (CP06), GFP and for NDUFS3 from Abcam (ab6556 and ab14711, respectively). Antibodies for ATFS-1 were previously described [5] . 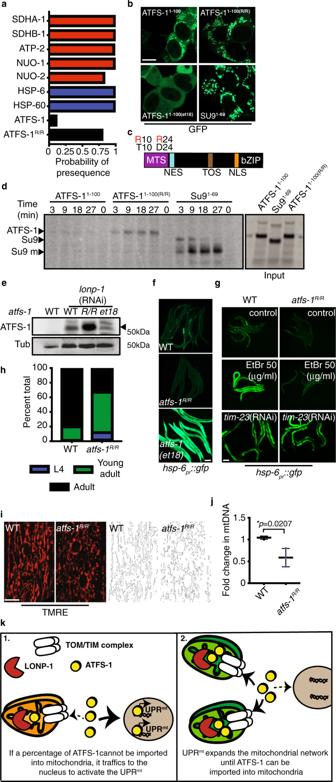Fig. 3: UPRmtrequires the weak MTS in ATFS-1. aMitochondrial targeting sequence probability prediction using MitoFates. OXPHOS proteins (red), mitochondrial chaperones (blue), ATFS-1 (black).bHEK293T cells expressing ATFS-11–100::GFP, ATFS-11-100(R/R)::GFP, ATFS-11-100(et18)::GFP or SU91–69::GFP. Scale bar 10 µm. Experiment was repeated two biologically independent times with similar results.cATFS-1 schematic highlighting ATFS-1R/Ramino acid substitutions.dIn organelle import of radiolabeled ATFS-11–100::GFP, ATFS-11-100(R/R)::GFP and Su91–69::GFP into isolated mitochondria. After the indicated time points, mitochondria were washed and analyzed by SDS-PAGE electrophoresis. ATFS-1, Su9, mature (m) are marked.N= 3 biologically independent experiments with similar results.eSDS-Page immunoblots of lysates from wild-type,atfs-1R/R, andatfs-1(et18)worms raised on control orlonp-1(RNAi). ATFS-1 is marked (‣) and tubulin (Tub) was used as a loading control.N= 3 biologically independent experiments with similar results.fhsp-6pr::gfpin wild-type,atfs-1(et18), andatfs-1R/Rworms. Scale bar 0.1 mm.N= 3 biologically independent experiments with similar results.ghsp-6pr::gfpin wild-type andatfs-1R/Rworms raised on 50 µg/ml EtBr, control, ortimm-23(RNAi). Scale bar 0.1 mm.N= 3 biologically independent experiments with similar results.hDevelopmental stages of 3-day-old wild-type oratfs-1R/Rworms.N= 158 worms (wild type) andN= 256 worms (atfs-1R/R). Experiments were repeated two biologically independent with similar results.iTMRE staining of wild-type andatfs-1R/Rworms. Skeleton-like binary backbone is presented (right). Scale bar 10 µm. Experiments were repeated three times with similar results.jQuantification of mtDNA in wild-type andatfs-1R/Rworms as determined by qPCR.N= 3 biologically independent experiments. Error bars mean ± SD (two-tailed Student’st-test).kProposed model for ATFS-1-mediated mitochondria expansion. Source data are provided as a Source Data file. 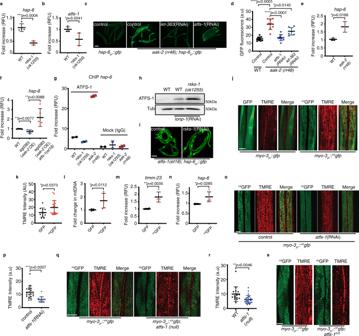Fig. 4: TORC1-mediated protein synthesis promotes ATFS-1 activation. a,bTranscript levels of heat shock protein-6 (hsp-6) (a) and of activated transcription factor stress-1 (atfs-1) (b) as determined by qRT-PCR in wild-type andrsks-1(ok1255)worms.N= 4 biologically independent experiments. Error bars mean ± SD (two-tailed Student’st-test). RFU, relative fluorescence units.chsp-6pr::gfpandaak-2(rr48);hsp-6pr::gfpworms raised on control,let-363, oratfs-1(RNAi). Scale bar 0.1 mm. Experiments were repeated three biologically independent times with similar results.dQuantification of GFP intensity inhsp-6pr::gfp(N= 10) andaak-2(rr48);hsp-6pr::gfpworms raised on control (N= 8 worms),let-363(N= 8 worms), oratfs-1(RNAi) (N= 7 worms). Error bars mean ± SD (two-tailed Student’st-test). a.u., arbitrary units.e,fTranscript levels of heat shock protein-6 (hsp-6) as determined by qRT-PCR in wild-type andaak-2(rr48)wormsN= 3 biologically independent experiments (e) and in wild type,agd383, andagd383;atfs-1(et18)strainsN= 5 biologically independent experiments (f). Error bars mean ± SD (two-tailed Student’st-test). RFU, relative fluorescence units.gChIP ofhsp-6promoter in wild-type,rsks-1(ok1255), andaak-2(rr48)worms as measured by qRT-PCR.N= 2 biologically independent experiments. RFU, relative fluorescence units.hSDS-Page immunoblots of wild-type andrsks-1(ok1255)worms, raised on control orlonp-1(RNAi). Tubulin (Tub) was used as a loading control.N= 3 biologically independent experiments with similar results.iatfs-1(et18);hsp-6pr::gfpworms raised on control orrsks-1(RNAi). Scale bar 0.1 mm. Experiments were repeated three biologically independent times with similar results.jTMRE staining (red) of worms expressingmyo-3pr::gfpormyo-3pr::mtgfp. Scale bar 10 µm. Experiments were repeated three biologically independent times with similar results.kQuantification of TMRE intensity in muscle cells of worms expressingmyo-3pr::gfpormyo-3pr::mtgfp.N= 34 worms (myo-3pr:: gfp),N= 24 worms (myo-3pr::mtgfp). Error bars mean ± SD (two-tailed Student’st-test). a.u., arbitrary units.lQuantification of mtDNA inmyo-3pr:: gfpandmyo-3pr::mtgfpworms as determined by qPCR.N= 6 biologically independent experiments. Error bars mean ± SD (two-tailed Student’st-test).m,nTranscript levels of translocase of inner mitochondrial membrane-23 (timm-23) (m) and of heat shock protein-6 (hsp-6) (n) as determined by qRT-PCR inmyo-3pr::gfpand inmyo-3pr::mtgfpworms.N= 4 biologically independent experiments. Error bars mean ± SD (two-tailed Student’st-test). RFU, relative fluorescence units.oTMRE staining of worms expressingmyo-3pr::mtgfpraised on control oratfs-1(RNAi). Scale bar 10 µm. Experiments were repeated three biologically independent times with similar results.pQuantification of TMRE intensity in muscle cells of worms expressingmyo-3pr::mtgfpraised on control oratfs-1(RNAi).N= 18 worms (control),N= 13 worms (atfs-1(RNAi)). Error bars mean ± SD (two-tailed Student’st-test). a.u., arbitrary units.qTMRE staining of wild-type andatfs-1(null) worms expressingmyo-3pr::mtgfp. Scale bar 10 µm. Experiments were repeated three biologically independent times with similar results.rQuantification of TMRE intensity in muscle cells of wild-type, andatfs-1(null)worms.N= 15 worms (wild type),N= 24 worms (atfs-1(null)). Error bars mean ± SD (two-tailed Student’st-test). a.u., arbitrary units.sTMRE staining of wild-type andatfs-1R/Rworms expressingmyo-3pr::mtgfp. Scale bar 10 µm. Experiments were repeated three biologically independent times with similar results. Source data are provided as a Source Data file. All antibodies were diluted 1 : 2000, except for ATFS-1, which was diluted 1 : 1000. Immunoblots were visualized using ChemiDoc XRS + system (Bio-Rad). All western blot experiments were performed at least three times. mtDNA quantification mtDNA quantification was performed using a quantitative PCR (qPCR)-based method similar to previously described assays [41] . Twenty to 30 worms were collected in 30 µl of lysis buffer (50 mM KCl, 10 mM Tris-HCl pH 8.3, 2.5 mM MgCl 2 , 0.45% NP-40, 0.45% Tween 20, 0.01% gelatin, with freshly added 200 µg/ml proteinase K) and frozen at −80 °C for 20 min prior to lysis at 65 °C for 80 min. Relative quantification was used for determining the fold changes in mtDNA between samples. 1 µl of lysate was used in each triplicate qPCR reaction. qPCR was performed using the Thermo Scientific SyBr Green Maxima Mix and the MyiQ2 Two-Color Real-Time PCR Detection System (Bio-Rad Laboratories). Primers that specifically amplify mtDNA are listed in Supplementary Data file 6 . Primers that amplify a non-coding region near the nuclear-encoded ges-1 gene were used as a control. mtDNA was harvested from synchronized worms at the L4 stage. All qPCR results have been repeated at least three times and performed in triplicates. A Student’s t -test was employed to determine the level of statistical significance. RNA isolation and qRT-PCR RNA isolation and quantitative reverse-transcriptase PCR (qRT-PCR) analysis were previously described [11] . Worms were synchronized by bleaching, raised on HT115 E. coli and harvested at the L4 stage. Total RNA was extracted from frozen worm pellets using RNA STAT (Tel-Test) and 500 ng RNA was used for cDNA synthesis with qScript™ cDNA SuperMix (QuantaBio). qPCR was performed using iQ™ SYBR® Green Supermix (Bio-Rad Laboratories). qPCR primers are listed in Supplementary Data file 6 . All qPCR results were repeated at least 3 times and performed in triplicates. A two-tailed Student’s t -test was employed to determine the level of statistical significance. Oxygen consumption Oxygen consumption was measured using a Seahorse XFe96 Analyzer at 25 °C similar to that described previously [42] . In brief, L4 worms were transferred onto empty plates and allowed to completely digest the remaining bacteria for 1 h, after which ten worms were transferred into each well of a 96-well microplate containing 180 µl M9 buffer. Basal respiration was measured for a total of 30 min, in 6 min intervals that included a 2 min mix, a 2 min time delay, and a 2 min measurement. To measure respiratory capacity, 15 µM carbonyl cyanide-4-(trifluoromethoxy)phenylhydrazone was injected, the oxygen consumption rate reading was allowed to stabilize for 6 min, then measured for five consecutive intervals. Mitochondrial respiration was blocked by adding 40 mM Sodium azide. Each measurement was considered one technical replicate. Cultured cells and imaging HEK293T cells were transfected with 0.5 µg of the expression plasmids: SU9 1–69 ::GFP with ATFS-1 1-100 ::GFP, ATFS-1 1-100(R/R) ::GFP, and ATFS-1 1-100(et18) ::GFP via Lipofectamine. The cells were imaged 16 h post transfection. RNA-seq and differential expression analysis cDNA libraries were constructed with standard Illumina P5 and P7 adapter sequences. The cDNA libraries were run on an Illumina HiSEq2000 instrument with single-read 50 bp. RNA reads were then aligned to WBcel235/ce11 reference genome and differential gene expression analysis was performed with edgeR [43] . Differences in gene expression between atfs-1(et18) and atfs-1(null) compared to wild type are listed in Supplementary Data files 7 and 8 , respectively. Data were deposited in GEO accession no. GSE114951 Analysis of worm development Worms were synchronized via bleaching and allowed to develop on HT115 bacteria plates for 3 days at 20 °C. Developmental stage was quantified as a percentage of the total number of animals. Each experiment was preformed three times. For the comparison of wild-type and atfs-1(null) worms; N = 162 (wild type), and 282 ( atfs-1(null) ). For the comparison of wild type to atfs-1 R/R worms; N = 158 (wild type) and N = 256 ( atfs-1 R/R ). Statistics All experiments were performed at least three times yielding similar results and comprised of biological replicates. The sample size and statistical tests were chosen based on previous studies with similar methodologies and the data met the assumptions for each statistical test performed. No statistical method was used in deciding sample sizes. No blinded experiments were performed, and randomization was not used. For all figures, the mean ± SD is represented unless otherwise noted. Prism 8 (GraphPad) is used for statistical analysis and graph creation. Microscopy C. elegans were imaged using either a Zeiss AxioCam 506 mono camera mounted on a Zeiss Axio Imager Z2 microscope or a Zeiss AxioCam MRc camera mounted on a Zeiss SteREO Discovery.V12 stereoscope. Images with high magnification (×63) were obtained using the Zeiss ApoTome.2. Exposure times were the same in each experiment. Cell cultures were imaged with the Zeiss LSM800 microscope. With the Zen 2.3 Blue software. All images are representatives of more than three images. Quantification of fluorescent intensity as well as creating binary skeleton-like structures were done with the Fiji software (Version 2.0.0-rc-69/1.52p) [44] . Gene set enrichment analysis The OXPHOS gene set was downloaded from WormBase Ontology Browser [45] . mRNA abundance was measured and ranked by reads per kilobase per million reads from RNA-seq data. Pre-ranked gene set enrichment analysis was performed with GSEA3.0 software with ‘classical’ scoring [46] . Transmission electron microscopy L4 larvae were transferred to 2.5% glutaraldehyde in 0.1 M Sodium Cacodylate buffer pH 7.2 for 10 min. The tail and head of each worm were dissected out and the main body was transferred to fresh 2.5% glutaraldehyde in 0.1 M Sodium Cacodylate buffer and kept at 4 °C overnight. Samples were processed and analyzed at the University of Massachusetts Medical School Electron Microscopy core facility according to standard procedures. Briefly, the samples were rinsed three times in the same fixation buffer and post-fixed with 1% osmium tetroxide for 1 h at room temperature. Samples were then washed three times with ddH 2 O for 10 min and then dehydrated through a graded ethanol series of 20% increments, before two changes in 100% ethanol. Samples were then infiltrated first with two changes of 100% Propylene Oxide and then with a 50%/50% propylene oxide/SPI-Pon 812 resin mixture. The following day, five changes of fresh 100% SPI-Pon 812 resin were performed before the samples were polymerized at 68 °C in flat pre-filled embedding molds. The samples were then reoriented, and thin sections (~70 nm) were placed on copper support grids and contrasted with Lead citrate and Uranyl acetate. Sections were examined using a CM10 TEM with 100 Kv accelerating voltage and images were captured using a Gatan TEM CCD camera. Ribosome profiling data analysis Ribosome profiling sequencing data were downloaded from the NCBI Sequence Read Archive (SRA) ( http://www.ncbi.nlm.nih.gov/sra/ ) under accession number SRA055804. Data were analyzed as previously described [30] . Data analysis was done with the help of Unix-based software tools. First, the quality of raw sequencing reads was determined by FastQC (version 0.11.9) [47] . Reads were then filtered according to quality via FASTQ for a mean Phred base calling quality score above 30 [48] . Filtered reads were mapped to the C. elegans reference genome (Wormbase WS275) using BWA (version 0.7.5) and SAM files were converted into BAM files by SAMtools (version 0.1.19). Coverage data for specific genes (including 5′-untranslated region (UTR), exons and 3′-UTR) were calculated by SAMtools and coverage data for each gene was plotted using R (version 3.5.2) [49] . Mitochondria isolation and in vitro protein import Cells (budding yeast W303) were grown to logarithmic phase in YPD (1% yeast extract, 2% peptone, 2% glucose), collected by centrifugation, and washed once with water. Cells were then resuspended in 0.1 M Tris pH 9.4, 10 mM dithiothreitol, and incubated for 20 min at 30 °C. Cell walls were disturbed by incubation in 1.2 M sorbitol, 20 mM K 2 HPO 4 pH 7.4, 1% zymolyase for 1 h at 30 °C. Dounce homogenization was used to lyse the cells in 0.6 M sorbitol, 10 mM Tris pH 7.4, 1 mM EDTA, fatty acid free 0.2% bovine serum albumin (BSA), and 1 mM phenylmethylsulfonyl fluoride (PMSF). Mitochondria were then isolated by differential centrifugation as described previously [50] and resuspended in SEM buffer (0.25 M sucrose, 10 mM MOPS-KOH pH 7.2, and 1 mM EDTA). The coupled Transcription/Translation system (T7 Quick for PCR DNA, Promega) was used to express ATFS-1 from a PCR template. Precursor proteins (ATFS-1 1–100 ::GFP, ATFS-1 1-100(R/R) ::GFP, and Su9 1–69 ::GFP) were synthesized in reticulocyte lysate in the presence of [35 S]methionine (T7 Quick for PCR DNA, Promega). Import into isolated mitochondria was performed in import buffer (3% (w/v) BSA, 250 mM sucrose, 80 mM KCl, 5 mM methionine, 5 mM MgCl 2 , 2 mM KH 2 PO 4 , 10 mM MOPS-KOH, pH 7.2, 4 mM NADH, 2 mM ATP, 5 mM creatine phosphate, 0.1 mg/ml creatine kinase) at 25 °C. The import reaction was stopped on ice or by addition of AVO (8 μM antimycin A, 20 μM oligomycin, 1 μM valinomycin). To dissipate Δψ, AVO was added before the import experiment. Samples were treated with 25 μg/ml proteinase K for 15 min on ice, following by treatment with 2 mM PMSF for 5 min on ice. Mitochondrial were washed twice with SEM buffer and analyzed by electrophoresis on SDS-polyacrylamide gel electrophoresis. The dried gel was exposed to a phospho screener, which was then scanned using a Typhoon Trio scanner (Amersham). Chromatin immunoprecipitation ChIP assays for ATFS-1 were performed as previously described [8] . Synchronized worms were cultured in liquid and harvested at early L4 stage by sucrose flotation. The worms were lysed via Teflon homogenizer in cold phosphate-buffered saline (PBS) with protease inhibitors (Roche). Cross-linking of DNA and protein was performed by treating the worms with 1.85% formaldehyde with protease inhibitors for 15 min. Glycine was added to a final concentration of 125 mM and incubated for 5 min at room temperature to quench the formaldehyde. The pellets were resuspended twice in cold PBS with protease inhibitors. Samples were sonicated in a Bioruptor (Diagenode) for 15 min at 4 °C on high intensity (30 s on and 30 s off). Samples were transferred to microfuge tubes and spun at 15,000 × g for 15 min at 4 °C. The supernatant was precleaned with pre-blocked ChIP-grade Pierce™ magnetic protein A/G beads (Thermo Scientific) and then incubated with ATFS-1 antibody or Mouse mAb IgG1 Isotype Control (Cell Signaling Technology, G3A1) rotating overnight at 4 °C. The antibody-DNA complex was precipitated with protein A/G magnetic beads or protein A sepharose beads (Invitrogen). After washing, the crosslinks were reversed by incubation at 65 °C overnight. The samples were then treated with RNaseA at 37 °C for 1.5 h followed by proteinase K at 55 °C for 2 h. Lastly, the immunoprecipitated and input DNA were purified with ChIP DNA Clean & Concentrator (Zymo Research, D5205) and used as templates for qPCR. Reporting summary Further information on research design is available in the Nature Research Reporting Summary linked to this article.